Three-photon bosonic coalescence in an integrated tritter The main features of quantum mechanics reside in interference deriving from the superposition of different quantum states. While current quantum optical technology enables two-photon interference both in bulk and integrated systems, simultaneous interference of more than two particles, leading to richer quantum phenomena, is still a challenging task. Here we report the experimental observation of three-photon interference in an integrated three-port directional coupler realized by ultrafast laser writing. By exploiting the capability of this technique to produce three-dimensional structures, we realized and tested in the quantum regime a three-port beam splitter, namely a tritter, which allowed us to observe bosonic coalescence of three photons. These results open new important perspectives in many areas of quantum information, such as fundamental tests of quantum mechanics with increasing number of photons, quantum state engineering, quantum sensing and quantum simulation. The Hong-Ou-Mandel effect is a purely quantum phenomenon deriving from the interference of two photons [1] . It is a consequence of the bosonic nature of light and it can be observed when two identical photons impinge simultaneously on a two-port balanced beam splitter and, as a result, they are forced to exit from the same port. This effect can be exploited to quantify the amount of indistinguishability of correlated photons [2] , [3] or to project a quantum state onto the maximally entangled singlet Bell state, representing an important resource in many research areas of quantum information, from quantum computation to quantum metrology [4] , [5] , [6] . The interaction of single-photon states on a beam splitter and successive post selection may indeed lead to the generation of entangled states [7] such as N00N and GHZ states [8] . As a matter of fact, achieving interference of more than two particles on a beam splitter is a challenging task [9] . However, it could open the door to the observation of quantum phenomena in increasing size systems and to the engineering of quantum states for quantum information processing [10] , [11] . The adoption of a multiport beam splitter has been proposed to perform additional classes of possible EPR-Bell experiments in a Hilbert space with dimension higher than two [12] . Furthermore the capability of implementing multipath interferometers by multiport beam splitters could be adopted to perform quantum computation tasks [13] . Recently a generalized N -port beam splitter has been theoretically addressed in [14] , [15] , and the behaviour of N photons impinging onto the N -port beam splitter has been studied by using a statistical approach, as the complexity of this problem grows faster than exponentially with growing N . Very recently, the application to quantum interferometry of three- and four-port beam splitters have been theoretically investigated, and a quantum enhancement in terms of sensitivity has been predicted [16] . However, three-particle interferometry is mostly unexplored territory, both experimentally and theoretically. The three-beam extension of a beam splitter, the so called ‘tritter’, was first addressed in [12] and its proposed implementation consisted of the combination of two-port beam splitters and phase shifters (see Fig. 1a ) ( [12] , [17] ). Three-dimensional implementations of three- and four-port beam splitters, based on fused optical fibres [18] or femtosecond laser waveguide writing [19] , [20] , [21] , have been proposed. However, only classical light or two-photon interference experiments were carried out on such devices. Therefore, an experimental investigation of quantum interference of more than two photons is still lacking. 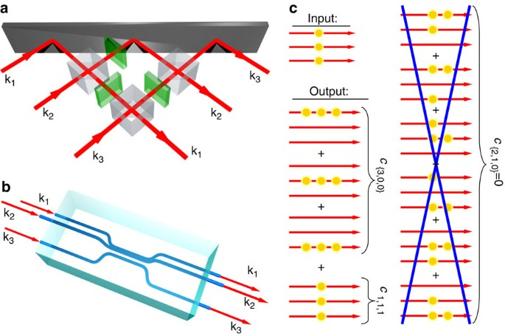Figure 1: Schematic representation of a tritter and related bosonic coalescence. (a) Optical scheme for a three-mode splitter obtained by a set of conventional beam splitters (grey cubes) and phase shifters (green plates)12,17, wherekiwithi=1,2,3 represent input–output spatial modes. (b) Integrated three-dimensional scheme for a laser-written tritter. (c) Three-photon bosonic coalescence effect in a tritter when each photon is injected into a different input spatial mode: all the terms with two photons exiting on the same output port vanish due to bosonic coalescence. Figure 1: Schematic representation of a tritter and related bosonic coalescence. ( a ) Optical scheme for a three-mode splitter obtained by a set of conventional beam splitters (grey cubes) and phase shifters (green plates) [12] , [17] , where k i with i =1,2,3 represent input–output spatial modes. ( b ) Integrated three-dimensional scheme for a laser-written tritter. ( c ) Three-photon bosonic coalescence effect in a tritter when each photon is injected into a different input spatial mode: all the terms with two photons exiting on the same output port vanish due to bosonic coalescence. Full size image Here we report the first experimental investigation of three-photon interference in a tritter. The tritter is realized by femtosecond laser waveguide writing and it consists of three waveguides approaching three-dimensionally, thus enabling simultaneous interaction of the three photons without having to decompose the process into cascaded two-mode interactions and phase shifters ( Fig. 1b ). The three photons, each coupled to a different waveguide, mutually interfere in the three-arm directional coupler by evanescent field interaction. The behaviour of a three-photon state entering the tritter is investigated by comparing the output state probabilities with the expected classical ones, evidencing the purely quantum effects involved in bosonic coalescence. Theoretical description of the tritter output probabilities Let us first address the action of a tritter on a generic input state | ψ ›. It can be expressed by a unitary matrix , mapping the input field operators to the output field operators with , ( [12] , [15] , [17] ; see Supplementary Note 1 ). In the case of an ideally symmetric tritter, where a photon entering in one input port has the same probability of exiting through anyone of the output ports, the unitary matrix reads: Let us consider what happens when an ideal tritter is injected by a three-photon state |1,1,1›. The corresponding output state after the evolution induced by reads: Here and , where |{ i , j , k }› is the symmetric superposition of the three-photon states corresponding to ( i , j , k ) photons exiting in the three output ports. We first observe that, as a consequence of bosonic coalescence, all the terms of two photons exiting from the same output port disappear ( Fig. 1c ). To fully describe three-photon interference we need to introduce two relative delays between the three bosons. We theoretically calculated the probability of the different output states [(1,1,1), (2,1,0), (3,0,0)] as a function of the relative delays x m = c τ m ( m =1, 2) between the three photons. These probabilities are represented in Fig. 2a–c as surfaces in a three-dimensional space and represent an extension of the well-known Hong-Ou-Mandel curves. This representation enables a deeper insight into three-photon interference, evidencing non-trivial features as a function of the two delays. In particular, we observe the presence of three regions: (i) the three input photons are indistinguishable when x 1 ~ x 2 ~0, this leads to a three-photon coalescence effect, resulting in a dip or a peak depending on the detected output state; (ii) only two of the three input photons are indistinguishable when x m ~0≠ x n or x m ~ x n ≠0; (iii) the three input photons are distinguishable when x 1 ≠ x 2 ≠0, leading to classically correlated outcomes. Here, the superscript q indicates the quantum nature of the three-photon coalescence, while the superscript cl highlights that the photons behave as classical particles. 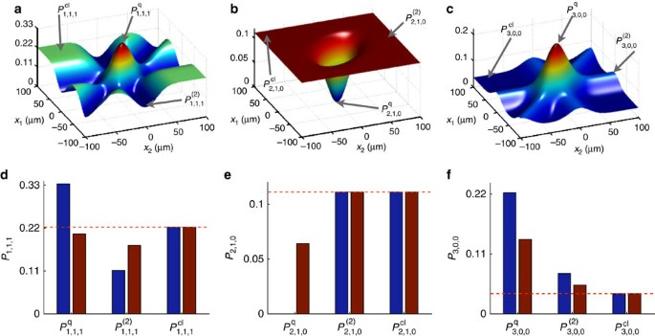Figure 2: Hong-Ou-Mandel effect for a |1, 1, 1› input state in an ideal tritter. Theoretical output probabilitiesP1,1,1(a),P2,1,0(b), andP3,0,0(c) as a function of the delaysxi=cτiof the impinging photons. (d–f) Theoretical output probabilitiesfor three indistinguishable input photons,for three photons out of interference andfor two indistinguishable and one delayed input photons. The red bars take into account the presence of partial distinguishability between the three impinging photons with indistinguishabilityp=0.65 whereas blue bars refer to perfectly indistinguishable photons withp=1 (seeSupplementary Note 4). The dashed horizontal lines represent the classical boundaries. Figure 2d–f compares the different probabilities corresponding to cases i–iii for each output state. Figure 2: Hong-Ou-Mandel effect for a |1, 1, 1› input state in an ideal tritter. Theoretical output probabilities P 1,1,1 ( a ), P 2,1,0 ( b ), and P 3,0,0 ( c ) as a function of the delays x i = c τ i of the impinging photons. ( d – f ) Theoretical output probabilities for three indistinguishable input photons, for three photons out of interference and for two indistinguishable and one delayed input photons. The red bars take into account the presence of partial distinguishability between the three impinging photons with indistinguishability p =0.65 whereas blue bars refer to perfectly indistinguishable photons with p =1 (see Supplementary Note 4 ). The dashed horizontal lines represent the classical boundaries. Full size image Tritter fabrication by ultrafast laser writing The tritter device was realized by adopting femtosecond laser-writing technology [22] , [23] , [24] . This technique exploits nonlinear absorption of focused femtosecond laser pulses that create permanent and localized increase of the refractive index in transparent materials. Waveguides are directly fabricated in the material bulk by translating the sample at constant speed along the desired path. This technique has the unique capability of producing integrated devices with three-dimensional geometries. Ultrafast laser-writing technique has rapidly become a powerful tool for demonstrating new quantum integrated devices, able to perform quantum logic operations [25] , as well as two-photon quantum walks [26] , [27] . The femtosecond laser-written tritter consists of three waveguides approaching and interacting in the coupling region ( Fig. 1b ). Thanks to this configuration equal coupling coefficients may be obtained, in a way that a single photon entering in any input port has the same probability to exit from any of the three output ports. This three-dimensional approach, enabled by femtosecond laser writing, avoids the use of cascaded beam splitters and phase shifters that are difficult to control and provides a compact device that can be effectively scaled in more complex architectures. Although conceptually simple, the tritter needs accurate dimensioning. As a first order arrangement, we consider the waveguides lying at the vertex of an equilateral triangle, where key parameters are waveguide spacing and length in the interaction region. Actually these two parameters are not independent as, in order to achieve an equal output distribution, the coupling coefficient k and interaction length L need to satisfy the relation kL =2 π /9 (see Supplementary Note 2 ). Sizing of the tritter starts from choosing the waveguide spacing d to the smallest value that avoids overlap (this will keep the device as short as possible). The chosen value of d in turn defines the coupling coefficient k and, thus, according to the previous relation, the interaction length L . However, the slightly elliptical-guided mode of the femtosecond laser-written optical waveguides and other fabrication imperfections require performing a second-order fine tuning of the device that can be accomplished by slightly shifting one of the three waveguides in a scalene triangle geometry. This fine tuning is performed most efficiently by an iterative procedure, where we take full advantage of the rapid prototyping capabilities of femtosecond laser waveguide writing (see Supplementary Fig. S1 for the final optimized geometry). Two-photon characterization of the tritter device To characterize the implemented device and to compare its unitary evolution with respect to the ideal case, we implemented the reconstruction method proposed in [28] . This technique consists in measuring all the possible two-photon Hong-Ou-Mandel interference fringes and then reconstructing the elements of the evolution matrix through a minimization procedure (see Supplementary Note 3 for more details). We show in Fig. 3 the real and imaginary parts of the reconstructed matrix at 795 nm wavelength, compared with the corresponding theoretical matrix . To quantify the quality of the fabrication process, we evaluated the similarity S between the two corresponding Hong-Ou-Mandel visibility matrices, defined as . The obtained value demonstrates a high correspondence of the implemented device with an ideal tritter. 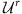Figure 3: Two-photon experimental reconstruction of the unitary matrixof the implemented tritter. Experimental two-photon Hong-Ou-Mandel interference for input states: (a) |1, 1, 0›, (b) |1, 0, 1› and (c) |0, 1, 1›. For each input state all possible output ones are acquired. Error bars in the experimental points are due to poissonian statistics of the measured signal. (d–e) Real and imaginary parts of. (f–g) Real and imaginary parts of the theoretical tritter. Figure 3: Two-photon experimental reconstruction of the unitary matrix of the implemented tritter. Experimental two-photon Hong-Ou-Mandel interference for input states: ( a ) |1, 1, 0›, ( b ) |1, 0, 1› and ( c ) |0, 1, 1›. For each input state all possible output ones are acquired. Error bars in the experimental points are due to poissonian statistics of the measured signal. ( d – e ) Real and imaginary parts of . ( f – g ) Real and imaginary parts of the theoretical tritter . Full size image Experimental three-photon interference We experimentally tested the three-photon coalescence by adopting the experimental setup shown in Fig. 4 . Four photons are produced by parametric down conversion: one of them acts as the trigger for coincidence detection, while the other three are coupled into the tritter, after passing through different delay lines. The output modes are detected by using optical fibre beam splitters and single-photon avalanche photodiodes. Coincidences between different detectors allow us to reconstruct the probability of obtaining a given output state. By changing the relative delays between the three photons, it is possible to observe the coalescence effects in the different experimental conditions, as shown in Fig. 2a–c . The tritter device, first characterized by single- and two-photon states at wavelength 795 nm (see Fig. 3 ) has then been tested by three photons at wavelength 785 nm, due to availability of higher transmissivity spectral filters at that wavelength. It has to be noted that the unitary matrix of the tritter at 785 nm is still in very good agreement with that of an ideal tritter (see equation 1), yielding a similarity (see Supplementary Note 3 and Supplementary Fig. S4 ). We have injected a three-photon state |1,1,1› and observed the different output contributions |1,1,1›, |2,1,0›, |3,0,0›. Due to the partial distinguishability between photons belonging to different pairs, the expected visibilities of peaks (or dips depending on the observed contributions) change depending on which photon is delayed. We compare in Fig. 5a the experimental and theoretical output states probabilities, obtained by delaying photons in different input modes for each measured output state. The expected probability values have been calculated by introducing in the theoretical model the distinguishability parameter p , which quantifies the distinguishability between the two different pairs, and by including six-photon events generated by the source. We investigated in Fig. 5b three-photon interference when delaying the partially distinguishable photon (case A in the figure) or when delaying one of the two indistinguishable ones (case B in the figure). In addition, we also considered the case when the partially distinguishable photon is kept out of the interference region and the two indistinguishable ones have a relative delay (case C in the figure). The latter case corresponds to two-photon interference although three photons are input and measured. It is observed that cases A and B are clearly different from case C. This demonstrates that the output states that we observe in cases A and B are indeed due to three-photon interference and cannot be attributed to two-photon interaction. To characterize whether the measured three-photon interference can be attributed to a quantum effect, we also compared the obtained visibilities with the classical bounds, calculated by injecting the tritter with three equal-amplitude coherent states with randomized phases [29] . We observe that the results obtained with the |1,1,1› input state outperform classical predictions, thus demonstrating the quantum origin of the measured three-photon interference. Details on the data analysis can be found in the Supplementary Note 4 . 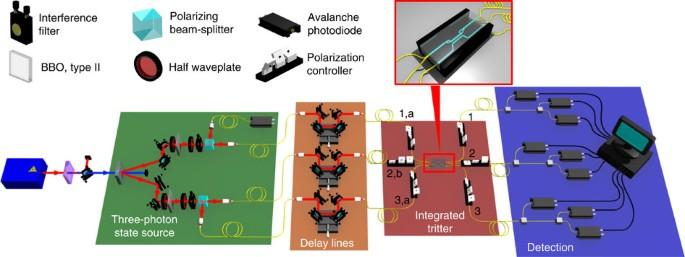Figure 4: Experimental layout. Experimental setup for the characterization of the tritter and the three-photon coalescence experiment. Two-photon and three-photon states, generated by parametric down conversion, are injected in the tritter device after the propagation through spatial delay lines. Then, coincidence detection at the output ports is performed to reconstruct the probability of obtaining a given output state realization (i,j,k). Labels 1, 2, 3 stand for spatial modes, while letter a refers to indistinguishable photons and b to the partially distinguishable one. BBO, β-barium borate crystal. Figure 4: Experimental layout. Experimental setup for the characterization of the tritter and the three-photon coalescence experiment. Two-photon and three-photon states, generated by parametric down conversion, are injected in the tritter device after the propagation through spatial delay lines. Then, coincidence detection at the output ports is performed to reconstruct the probability of obtaining a given output state realization ( i , j , k ). Labels 1, 2, 3 stand for spatial modes, while letter a refers to indistinguishable photons and b to the partially distinguishable one. BBO, β-barium borate crystal. 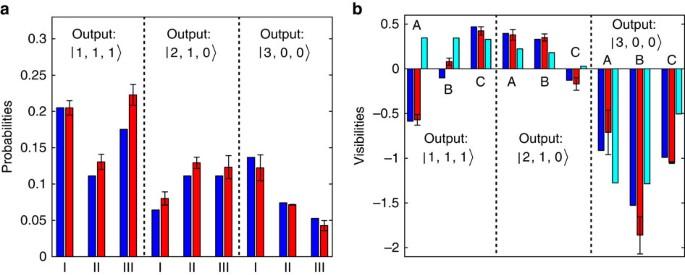Figure 5: Experimental results with a three-photon input state. (a) Output probabilities for different choices of the delayed photon and of the measured output state contribution. Case I: three-photon interference. Case II: distinguishable photon on input port 2 delayed (two-photon interference). Case III: identical photon on input port 3 delayed (two-photon interference). Blue bars: theoretical prediction obtained from the reconstructed tritter matrixand partially distinguishable photon pairs. Red bars: experimental results. (b) VisibilitiesV=(Γ∞–Γ0)/Γ∞for different choices of the delayed photon and of the measured output state contribution. Here, Γ∞and Γ0correspond respectively to the number of four-fold coincidences when the delayed photon is, respectively, out or inside the interference region. Case A: distinguishable photon on input port 2 delayed (three-photon interference). Case B: identical photon on input port 3 delayed (three-photon interference). Case C: distinguishable photon on input port 2 out of interference region and identical photon on input port 3 delayed (two-photon interference). Blue bars: theoretical prediction obtained from the reconstructed tritter matrixand partially distinguishable photon pairs. Red bars: experimental results. Cyan bars: expected visibilities with classical states. Error bars are due to poissonian statistics of the measured signal. Full size image Figure 5: Experimental results with a three-photon input state. ( a ) Output probabilities for different choices of the delayed photon and of the measured output state contribution. Case I: three-photon interference . Case II: distinguishable photon on input port 2 delayed (two-photon interference) . Case III: identical photon on input port 3 delayed (two-photon interference) . Blue bars: theoretical prediction obtained from the reconstructed tritter matrix and partially distinguishable photon pairs. Red bars: experimental results. ( b ) Visibilities V =(Γ ∞ –Γ 0 )/Γ ∞ for different choices of the delayed photon and of the measured output state contribution. Here, Γ ∞ and Γ 0 correspond respectively to the number of four-fold coincidences when the delayed photon is, respectively, out or inside the interference region. Case A: distinguishable photon on input port 2 delayed (three-photon interference). Case B: identical photon on input port 3 delayed (three-photon interference). Case C: distinguishable photon on input port 2 out of interference region and identical photon on input port 3 delayed (two-photon interference). Blue bars: theoretical prediction obtained from the reconstructed tritter matrix and partially distinguishable photon pairs. Red bars: experimental results. Cyan bars: expected visibilities with classical states. Error bars are due to poissonian statistics of the measured signal. Full size image We reported on the experimental observation of three-photon bosonic coalescence effect occurring within an integrated, three-dimensional, three-port beam splitter realized by the ultrafast laser-writing technique. To the best of our knowledge, this result represents the first experimental observation of the bosonic coalescence of three indistinguishable photons in a symmetric three-port device. The intrinsically stable and compact nature of this device makes it a fundamental building block for future complex networks implemented by integrated optical circuits. These devices are expected to open new perspectives in many research areas of quantum information. Indeed, the N -port beam splitters may find a wide range of applications in both quantum interferometry and quantum metrology. A first theoretical analysis performed in [16] shows that these devices can be exploited to build N -mode interferometers, where the adoption of quantum input states can lead to a significant enhancement in phase estimation protocols. Furthermore, the capability of conditionally generating path-entangled states may be increased by adopting structures composed of N -port beam splitters rather than conventional two-mode couplers [30] . This is expected to lead to a corresponding reduction in complexity of the experimental schemes in terms of the number of optical elements. Several other contexts may benefit from the adoption of N -port beam splitters. For instance, they can be adopted for the realization of ‘proof-of-principle’ quantum simulators [31] , and, combined in a modular structure, they can be used to realize full-scale quantum simulators for large-size quantum systems. The adoption of multiphoton-multimode platforms may indeed disclose the ‘hard-to-simulate’ scenario by adopting linear optics to implement a computational power beyond the one of a classical computer [32] . Furthermore, the development of complex integrated quantum devices may lead to implement fundamental tests of quantum mechanics, such as nonlocality tests, for quantum systems of increasing dimensionality [33] . Waveguide fabrication Waveguides are directly written in borosilicate glass substrate (EAGLE2000, Corning Inc.) using a cavity-dumped Yb:KYW oscillator, which provides 300 fs pulses at 1 MHz repetition rate. The laser beam is focused, by a 0.6-NA × 50 microscope objective, at 170 μm (average) depth under the glass surface. Optimum irradiation parameters for single-mode waveguiding at 795 nm wavelength are 220 nJ pulse energy and 40 mm/s translation speed. Sample translation at uniform speed is provided by high precision, three-axis air-bearing stages (Aerotech FiberGlide3D, Aerotech Inc.). The produced tritter is subsequently pigtailed by bonding fibre arrays on both sides of the device in order to obtain a compact and portable device. Four-photon source and detection apparatus Let us refer to the experimental setup shown in Fig. 4 in the main text. A 2-mm-thick β-barium borate crystal cut for type-II phase matching is pumped by the second harmonic of a Ti:sapphire mode-locked laser beam, and generates via spontaneous parametric down conversion at second-order two polarization photon pairs over two different spatial modes. The four photons [34] , [35] of the generated state are spectrally filtered by interferential filters (wavelength λ= 785 nm, Δ λ= 3 nm) and selected by four single-mode fibres placed at the output of two polarizing beam splitters. The spatial and temporal walk-off is compensated by inserting a waveplate and a 1-mm thick β-barium borate crystal crystal on each spatial mode. One of the four photons is detected to work as the trigger of the experiment. The other three photons are injected each into a single-mode fibre and, after passing through three delay lines and after polarization compensation, are coupled inside the tritter device. The output modes are sent to the detection stage. Four-fold coincidence detections are measured. The |1,1,1› contribution is measured by directly sending each output mode to a single-photon detector. The |2,1,0› (|3,0,0›) contribution is measured by splitting mode 1 in two (three) equal parts by means of fibre beam splitters and by placing a single-photon detector on each of the two (three) outputs of the fibre beam splitter system. The efficiencies for the three schemes including the trigger detector are respectively η 4 , (2/3) η 4 and (2/9) η 4 , being η the quantum efficiency of a single detector. How to cite this article: Spagnolo, N. et al. Three-photon bosonic coalescence in an integrated tritter. Nat. Commun. 4:1606 doi: 10.1038/ncomms2616 (2013).